Recruitment of mesenchymal stem cells into prostate tumours promotes metastasis Tumours recruit mesenchymal stem cells to facilitate healing, which induces their conversion into cancer-associated fibroblasts that facilitate metastasis. However, this process is poorly understood on the molecular level. Here we show that CXCL16, a ligand for CXCR6, facilitates mesenchymal stem cell or very small embryonic-like cells recruitment into prostate tumours. CXCR6 signalling stimulates the conversion of mesenchymal stem cells into cancer-associated fibroblasts, which secrete stromal-derived factor-1, also known as CXCL12. CXCL12 expressed by cancer-associated fibroblasts then binds to CXCR4 on tumour cells and induces an epithelial-to-mesenchymal transition, which ultimately promotes metastasis to secondary tumour sites. Our results provide the molecular basis for mesenchymal stem cell recruitment into tumours and how this process leads to tumour metastasis. Tumours have long been considered as wounds that do not heal [1] . Wound healing normally requires the participation of many different cell types as well as the activation of a vast number of cellular processes including matrix degradation, proliferation and recruitment of inflammatory cells. In addition, cells such as fibroblasts, epithelial and endothelial cells are also recruited and they too must coordinate their activities with inflammatory cells to pattern regeneration of normal tissues. As in normal wound healing, tumours also activate the recruitment of host cells into tumour beds to regulate survival and proliferation [2] . In this context, recent attention has focused on the roles of dendritic, tumour-associated macrophages and other early hematopoietic lineage populations that establish niches within tumours that foster and protect cancer stem cells from cytotoxic and metabolic stresses [3] . Moreover, many of these same cell populations are thought to promote and establish premetastatic niches at distant sites, which ultimately facilitate the ability of disseminated tumour cells to establish metastatic foci [4] , [5] . Mesenchymal stem cells (MSCs) are multipotent cells that contribute to tissue homoeostasis and regeneration. Normally, MSCs are rapidly recruited into sites of injury and inflammation where they differentiate into a variety of connective tissue cell types [6] , [7] . Recently, marrow-derived MSCs were shown to participate in tumour progression by establishing a favourable tumour microenvironment, differentiating into cancer-associated fibroblasts (CAFs), which establish cytokine networks that promote progression and migration [8] , [9] , [10] , [11] , [12] , [13] . Precisely how MSCs are recruited into primary tumour sites, how they contribute to the development of tumour niches for cancer stem cells, what regulates the conversion of MSCs into CAFs and how CAFs promote metastasis is not entirely understood. Skeletal metastases are one of the most serious complications of prostate cancer [14] . Growing evidence suggests that the CXC chemokine ligand 16 (CXCL16) and its receptor CXCR6 have important roles in tumour progression and bone metastasis [15] , [16] , [17] , [18] . CXCL16 is one of a small number of chemokines expressed as both soluble and cell surface molecules and it functions as a chemoattractant for many cell types [19] . CXCL16 is secreted by cells in response to IFN-γ, TNF-α and IL-1β (refs 18 , 20 , 21 , 22 , 23 , 24 , 25 , 26 ). CXCL16 is the sole ligand for CXCR6, a member of the seven transmembrane G protein-coupled receptor family, which signals through the AKT/mTOR pathways [16] . Our group has shown that in primary and metastatic prostate cancer, CXCL16 is highly expressed compared with normal prostate epithelial cells [16] , [27] . In addition, CXCL16/CXCR6 is involved in prostate cancer migration and invasion [16] , [19] , [24] , [27] . In the present study we demonstrate that tumour growth is dependent on the recruitment of MSCs into human and mouse prostate cancer in response to CXCL16. Once in the tumour, CXCL16 binding to CXCR6 expressed by MSCs, stimulates their conversion into CAFs, which subsequently secrete enhanced levels of CXCL12. CXCL12 expression by CAFs promotes an epithelial-to-mesenchymal transition (EMT) of the cancer cells, which supports metastasis to secondary sites. Together, these studies provide the molecular basis for MSC recruitment into primary tumours, and the conversion of MSCs into CAFs that ultimately lay the foundations for the EMT required for establishing distant metastasis. CXCL16 secreted by prostate cancer recruits MSCs We reasoned that cells with stem cell-like properties must rapidly migrate into wounds to initiate tissue regeneration. We hypothesized that CXCR6-expressing MSCs from the bone marrow are likely rapidly recruited into tumours in response to CXCL16. Therefore, human and mouse bone marrow MSCs ( Supplementary Fig. S1a ) were evaluated for CXCR6 expression. Human ( Fig. 1a ) and freshly isolated non-passaged (P 0 ) murine MSCs (Lin − Sca-1 + CD45 − or very small embryonic-like (VSEL) stem cells) [7] , [28] , [29] and second passage MSCs (P 2 ) expressed CXCR6, while MSCs isolated from CXCR6 −/− (MSC CXCR6 −/− ) mice did not ( Fig. 1c ). Tissue microarrays from prostate cancer patients demonstrated that CXCL16 expression correlated with tumour aggressiveness ( Fig. 1e ; Supplementary Fig. S1b ). Prostate cancer and breast cancer cell lines expressed significant levels of CXCL16 ( Fig. 1f ; Supplementary Fig. S1c–g ). In vitro , P 0 or P 2 MSCs isolated from CXCR6 wild-type mice (MSC CXCR6+/+ ) migrated towards CXCL16, while MSC CXCR6−/− did not ( Fig. 1h ). To determine what role CXCL16 has in recruiting MSCs into tumours, prostate cancer was implanted subcutaneously (s.c.) into CXCR6 +/+ or CXCR6 −/− mice ( Supplementary Fig. S1h ). Significantly, greater tumour volume was observed when the tumours were grown in CXCR6 +/+ versus CXCR6 −/− mice, suggesting that CXCR6-expressing host cells modulate tumour growth ( Fig. 1i ). Surprisingly, more MSCs were found in the tumours grown in the CXCR6 +/+ mice than in the tumours grown in CXCR6 −/− mice ( Fig. 1j ; Supplementary Table S1 ), though there were no differences in MSC numbers in the marrow of the CXCR6 +/+ versus CXCR6 −/− mice ( Supplementary Fig. S1i ), suggesting a specific recruitment of MSCs into tumours facilitates growth. 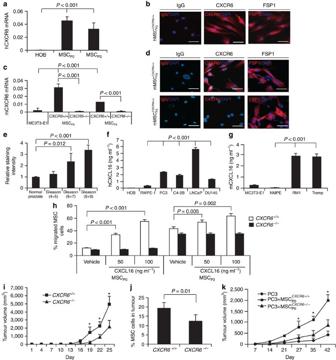Figure 1: Expression of CXCL16 by prostate cancer recruits MSCs into tumours to support tumour growth. (a) CXCR6 mRNA expression by human MSCs (P0and P2). (b) Expression of CXCR6 protein by human MSCs. Controls included isotype-matched antibodies and fibroblast-specific protein 1 (FSP1) for MSCs. Scale bars, 100 μm. (c) CXCR6 mRNA by mMSCs. CXCR6 expression was determined in freshly isolated, non-cultured (P0) or P2murine MSCs fromCXCR6+/+orCXCR6−/−mice. Human and murine osteoblasts (HOB and MC3T3-E1) were used as a negative control. (d) Expression of CXCR6 by murine P2CXCR6+/+orCXCR6−/−MSCs by immunohistochemistry (IHC) staining. Scale bar, 100 μm. Data ina–care representative of mean with s.d. for triplicates in each of the three independent experiments (Student’st-test). (e) CXCL16 expression in human prostate cancer tissue microarray inSupplementary Fig. S1b. Differences noted between normal prostate (n=30), Gleason 4+5 (n=9), Gleason 6+7 (n=18), and Gleason 8+9 (n=15) (mean±s.d. Student’st-test). Secretion of CXCL16 by human prostate cancer cell lines (f) and murine prostate cancer cell lines (g) as determined by ELISA (mean±s.d.,n=3 independent experiments, Student’st-test). (h) Migration of freshly isolated, non-cultured (P0) or P2murine MSCs fromCXCR6+/+orCXCR6−/−mice in response to CXCL16. The % migrated MSC was determined by hemocytometer counting (mean±s.d.,n=3 independent experiments, Student’st-test). (i)CXCR6+/+orCXCR6−/−mice were implanted s.c. with RM1 cells and caliper measurements of tumour growth performed over 25 days. *Significant differences between tumours grownCXCR6+/+andCXCR6−/−mice (mean±s.d., for 7 animals per group,n=3 independent experiments,P<0.05; Student’st-test). (j) % MSCs (P0) present in RM1 tumours grown inCXCR6+/+orCXCR6−/−mice at day 25 (mean±s.d. for 7 animals per group,n=3 independent experiments, Student’st-test). (k) SCID mice were implanted s.c. with PC3 cells mixed with MSCP0CXCR6+/+or MSCP0CXCR6−/−cells and tumour growth was evaluated by caliper measurements over 42 days. *Significant differences between tumours grown with PC3 cells mixed with MSCP0CXCR6+/+and MSCP0CXCR6−/−cells (mean±s.d. forn=5 animals per group,n=1 independent experiment,P<0.05, Student’st-test). Figure 1: Expression of CXCL16 by prostate cancer recruits MSCs into tumours to support tumour growth. ( a ) CXCR6 mRNA expression by human MSCs (P 0 and P 2 ). ( b ) Expression of CXCR6 protein by human MSCs. Controls included isotype-matched antibodies and fibroblast-specific protein 1 (FSP1) for MSCs. Scale bars, 100 μm. ( c ) CXCR6 mRNA by mMSCs. CXCR6 expression was determined in freshly isolated, non-cultured (P 0 ) or P 2 murine MSCs from CXCR6 +/+ or CXCR6 −/− mice. Human and murine osteoblasts (HOB and MC3T3-E1) were used as a negative control. ( d ) Expression of CXCR6 by murine P 2 CXCR6 +/+ or CXCR6 −/− MSCs by immunohistochemistry (IHC) staining. Scale bar, 100 μm. Data in a – c are representative of mean with s.d. for triplicates in each of the three independent experiments (Student’s t -test). ( e ) CXCL16 expression in human prostate cancer tissue microarray in Supplementary Fig. S1b . Differences noted between normal prostate ( n =30), Gleason 4+5 ( n =9), Gleason 6+7 ( n =18), and Gleason 8+9 ( n =15) (mean±s.d. Student’s t -test). Secretion of CXCL16 by human prostate cancer cell lines ( f ) and murine prostate cancer cell lines ( g ) as determined by ELISA (mean±s.d., n =3 independent experiments, Student’s t -test). ( h ) Migration of freshly isolated, non-cultured (P 0 ) or P 2 murine MSCs from CXCR6 +/+ or CXCR6 −/− mice in response to CXCL16. The % migrated MSC was determined by hemocytometer counting (mean±s.d., n =3 independent experiments, Student’s t -test). ( i ) CXCR6 +/+ or CXCR6 −/− mice were implanted s.c. with RM1 cells and caliper measurements of tumour growth performed over 25 days. *Significant differences between tumours grown CXCR6 +/+ and CXCR6 −/− mice (mean±s.d., for 7 animals per group, n =3 independent experiments, P <0.05; Student’s t -test). ( j ) % MSCs (P 0 ) present in RM1 tumours grown in CXCR6 +/+ or CXCR6 −/− mice at day 25 (mean±s.d. for 7 animals per group, n =3 independent experiments, Student’s t -test). ( k ) SCID mice were implanted s.c. with PC3 cells mixed with MSC P0 CXCR6+/+ or MSC P0 CXCR6 −/− cells and tumour growth was evaluated by caliper measurements over 42 days. *Significant differences between tumours grown with PC3 cells mixed with MSC P0 CXCR6+/+ and MSC P0 CXCR6 −/− cells (mean±s.d. for n =5 animals per group, n =1 independent experiment, P <0.05, Student’s t -test). Full size image To validate that these results were representative of other tumours and not specific to subcutaneous tumour growth, the studies were repeated with human prostate cancer and breast cancer cell lines in an orthotopic setting. As seen previously, robust MSC recruitment into the tumours occurred when prostate cancer or breast cancer cell lines were implanted in an orthotopic setting ( Supplementary Fig. S1j–r ; Supplementary Table S1 ). To confirm that MSCs signalling through CXCR6 has a critical role in tumour growth, prostate cancer cells were mixed with MSC P0 CXCR6+/+ or MSC P0 CXCR6 −/− and tumour growth was monitored. As predicted, significantly larger tumour growth occurred when the tumour cells were mixed with MSCs expressing CXCR6 (MSC P0 CXCR6+/+ ) compared with tumours established with MSCs not in which CXCR6 expression is knocked out (MSC P0 CXCR6 −/− ) ( Fig. 1k ). Together these findings suggest a key role for CXCL16/CXCR6 in recruiting MSCs into tumours, and supporting tumour growth. CXCL16/CXCR6 signalling induces CAF formation and CXCL12 Local and recruited MSCs are known to convert into tumour-associated fibroblasts (TAFs) or CAFs in close proximity to tumour cells [30] , [31] . To test whether prostate cancer-derived CXCL16 facilitates the conversion of MSCs into CAFs, MSCs were treated with CXCL16 and examined for expression of α-SMA and vimentin. MSCs CXCR6+/+ converted to α-SMA + and vimentin + expressing cells after CXCL16 stimulation, while MSCs CXCR6 −/− did not ( Fig. 2a–d ). To further investigate the role that CXCL16/CXCR6 signalling has in tumour growth, MSCs isolated from CXCR6 +/+ or CXCR6 −/− mice were treated with conditioned media derived from human and murine prostate cancer cell lines and examined for expression of α-SMA and vimentin. MSC CXCR6+/+ cells expressed significant levels of α-SMA and vimentin after treatment with conditioned media derived from prostate cancer cell lines, while MSC CXCR6 −/− cells did not ( Fig. 2e ; Supplementary Fig. S2a,b ). To validate these observations, prostate tumours grown in CXCR6 +/+ or CXCR6 −/− mice were probed for the CAF phenotype ( Supplementary Fig. S2c ). Paralleling the in vitro findings, fewer α-SMA + and vimentin + cells were identified in tumours grown in the CXCR6 −/− mice compared with CXCR6 +/+ mice ( Fig. 2g ). Previously, we demonstrated that CXCL16 expression in human tumours corresponds with increasing Gleason grade [27] . Therefore, to validate the murine observations in a human setting, tumour tissue microarrays derived from human prostate cancer samples were stained for vimentin. The data demonstrate that more CAFs expressing vimentin were detected in the Gleason 4+5 prostate cancer than in the benign prostate cancer tissues ( Fig. 2h ; Supplementary Fig. S2d ). A second critical feature of the CAF phenotype is the expression of stromal-derived factor-1 (SDF-1 or CXCL12), which facilitates metastases [32] , [33] . Colocalization studies identified that more α-SMA + /CXCL12 + and vimentin + /CXCL12 + -expressing cells were observed in tumours isolated from CXCR6 +/+ versus CXCR6 −/− mice ( Fig. 2j ) and greater levels of CXCL12 were identified in the extracellular milieu of tumours grown in CXCR6 +/+ versus CXCR6 −/− mice ( Fig. 2l ) or when mMSCs are treated with CXCL16 (Supplementary Fig. S2e). Next, CXCL12 secretion by MSCs was examined in response to CXCL16. MSC CXCR6+/+ but not MSCs CXCR6 −/− secreted CXCL12 in response to CXCL16 ( Fig. 2m ), which was regulated through Erk and NF-κB signalling ( Supplementary Fig. S2f–h ). 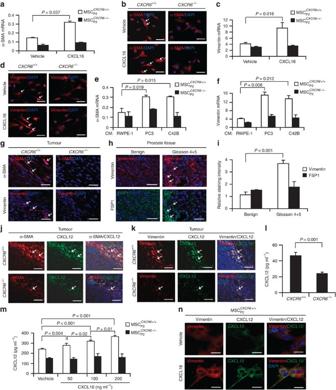Figure 2: Expression of CXCL12 by CAFs is dependent on CXCL16/CXCR6. MSCs isolated from CXCR6+/+or CXCR6−/−mice (P2) were exposed to vehicle or CXCL16 (100 ng ml−1) for 7 days. The expression of α-SMA (a) mRNA by qRT–PCR or (b) protein by immunohistochemistry (IHC) (red, α-SMA, white arrows; blue, DAPI nuclear stain), or for vimentin (c) mRNA or (d) protein (red, vimentin, white arrows; blue, DAPI nuclear stain) were evaluated. Scale bars, 100 μm. MSCs isolated fromCXCR6+/+orCXCR6−/−mice were exposed to human prostate cancer cell conditioned media for 7 days. The expression of α-SMA (e) and vimentin (f) mRNA were evaluated by qRT–PCR. (g) IHC of localization of α-SMA and vimentin-positive cells within tumours grown inCXCR6+/+orCXCR6−/−mice (red, α-SMA or vimentin, white arrow; blue, DAPI nuclear stain). Scale bars, 100μm. Data ina,c,eandfare representative of mean with s.d. for triplicates in each of the three independent experiments (Student’st-test). (h) IHC of vimentin or FSP1-positive cells within benign or Gleason 4+5 prostate cancers in human tissue microarrays (TMAs) (red, vimentin, white arrows; green, FSP1,white arrows; blue, DAPI nuclear stain). Staining for FSP1 served as a positive control of MSCs. Scale bars, 100 μm. (i) Quantification ofFig. 2h. Mean expression scores were multiplied by percent of positive cells in the field. Significant differences were noted between benign (n=30) or Gleason 4+5 prostate (n=6) (mean±s.d., Student’st-test). Colocalization of CXCL12 expression with (j) α-SMA- and (k) vimentin-positive cells (white arrows) within tumours grown inCXCR6+/+orCXCR6−/−mice. Scale bars, 100 μm. (l) CXCL12 protein expression in the extracellular milieu within tumours grown inCXCR6+/+orCXCR6−/−mice (mean±s.d., for triplicates in each of three independent experiments, Student’st-test). (m) Secretion of CXCL12 from MSCP2CXCR6+/+cells or MSCP2CXCR6−/−cells were observed following exogenous CXCL16 treatment by ELISA (mean±s.d. for triplicates in each of three independent experiments, Student’st-test, analysis of variance). (n) Colocalization of CXCL12 with vimentin following exposure of MSCP2CXCR6+/+cells or MSCP2CXCR6−/−cells to CXCL16in vitro. Scale bars, 100 μm. Figure 2: Expression of CXCL12 by CAFs is dependent on CXCL16/CXCR6. MSCs isolated from CXCR6 +/+ or CXCR6 −/− mice (P 2 ) were exposed to vehicle or CXCL16 (100 ng ml −1 ) for 7 days. The expression of α-SMA ( a ) mRNA by qRT–PCR or ( b ) protein by immunohistochemistry (IHC) (red, α-SMA, white arrows; blue, DAPI nuclear stain), or for vimentin ( c ) mRNA or ( d ) protein (red, vimentin, white arrows; blue, DAPI nuclear stain) were evaluated. Scale bars, 100 μm. MSCs isolated from CXCR6 +/+ or CXCR6 −/− mice were exposed to human prostate cancer cell conditioned media for 7 days. The expression of α-SMA ( e ) and vimentin ( f ) mRNA were evaluated by qRT–PCR. ( g ) IHC of localization of α-SMA and vimentin-positive cells within tumours grown in CXCR6 +/+ or CXCR6 −/− mice (red, α-SMA or vimentin, white arrow; blue, DAPI nuclear stain). Scale bars, 100μm. Data in a , c , e and f are representative of mean with s.d. for triplicates in each of the three independent experiments (Student’s t -test). ( h ) IHC of vimentin or FSP1-positive cells within benign or Gleason 4+5 prostate cancers in human tissue microarrays (TMAs) (red, vimentin, white arrows; green, FSP1,white arrows; blue, DAPI nuclear stain). Staining for FSP1 served as a positive control of MSCs. Scale bars, 100 μm. ( i ) Quantification of Fig. 2h . Mean expression scores were multiplied by percent of positive cells in the field. Significant differences were noted between benign ( n =30) or Gleason 4+5 prostate ( n =6) (mean±s.d., Student’s t -test). Colocalization of CXCL12 expression with ( j ) α-SMA- and ( k ) vimentin-positive cells (white arrows) within tumours grown in CXCR6 +/+ or CXCR6 −/− mice. Scale bars, 100 μm. ( l ) CXCL12 protein expression in the extracellular milieu within tumours grown in CXCR6 +/+ or CXCR6 −/− mice (mean±s.d., for triplicates in each of three independent experiments, Student’s t -test). ( m ) Secretion of CXCL12 from MSC P2 CXCR6+/+ cells or MSC P2 CXCR6 −/− cells were observed following exogenous CXCL16 treatment by ELISA (mean±s.d. for triplicates in each of three independent experiments, Student’s t -test, analysis of variance). ( n ) Colocalization of CXCL12 with vimentin following exposure of MSC P2 CXCR6+/+ cells or MSC P2 CXCR6 −/− cells to CXCL16 in vitro . Scale bars, 100 μm. Full size image Knockdown of CXCL16 reduces MSC recruitment and CAF formation To further explore the role of CXCL16 secreted by tumour cells and MSC cell recruitment, lentiviral vectors were used to silence CXCL16 expression in RM1 cells (RM1 shCXCL16 ). After clonal selection, individual clones were pooled and assayed by qRT–PCR and ELISA for the reduction of CXCL16 expression ( Fig. 3a ). We then tested whether RM1 shCXCL16 cells have the same capabilities to stimulate migration of MSCs compared with control (RM1 Control ) cells. As expected, the knockdown of CXCL16 expression in RM1 cells inhibited the migration of MSC cells in vitro ( Fig. 3c ). In conjunction with these studies, tumour growth over time was evaluated in CXCR6 +/+ mice ( Fig. 3d ). As shown in Fig. 3e , tumours generated from the RM1 Control cells rapidly developed, while tumour growth of the RM1 shCXCL16 cells was dramatically suppressed. Importantly, more P 0 MSCs were identified in the tumours grown with RM1 Control cells than in tumours grown with RM1 shCXCL16 cells ( Fig. 3f ; Supplementary Table S1 ). Taken together, these data suggest that CXCL16 expression by prostate tumours is critical for tumour growth and MSC cell recruitment. 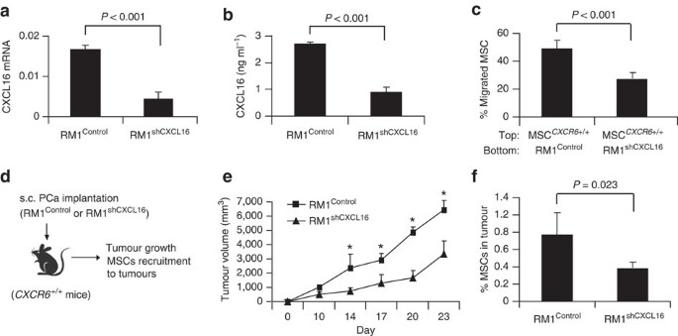Figure 3: Knockdown of prostate cancer cells reduces the tumour growth and MSC cell recruitment. (a) Expression of CXCL16 mRNA in the RM1Controlor RM1shCXCL16cells by qRT–PCR. (b) Secretion of CXCL16 by RM1Controlor RM1shCXCL16cells was determined by ELISA. (c) Migration of MSCCXCR6+/+cells was determined towards RM1Controlcells or RM1shCXCL16cells. Data ina–care representative of mean with s.d. for triplicates in each of three independent experiments (Student’st-test). Significance was determined using a Student’st-test. (d) Experimental scheme of RM1Controlor RM1shCXCL16cell implantation toCXCR6+/+mice for examining tumour growth and MSC cell recruitment to tumours. (e) The tumour growth of RM1Controlor RM1shCXCL16cells onCXCR6+/+mice was evaluated by caliper measurements over 23 days. *Significant differences between tumours grown with RM1Controland RM1shCXCL16cells (mean±s.d., forn=5 animals per group,n=2 independent experiments,P<0.05; analysis of variance). (f) % MSCs present in RM1Controlor RM1shCXCL16tumours grown inCXCR6+/+mice (mean±s.d., forn=5 animals per group,n=2 independent experiments, Student’st-test). Figure 3: Knockdown of prostate cancer cells reduces the tumour growth and MSC cell recruitment. ( a ) Expression of CXCL16 mRNA in the RM1 Control or RM1 shCXCL16 cells by qRT–PCR. ( b ) Secretion of CXCL16 by RM1 Control or RM1 shCXCL16 cells was determined by ELISA. ( c ) Migration of MSC CXCR6+/+ cells was determined towards RM1 Control cells or RM1 shCXCL16 cells. Data in a – c are representative of mean with s.d. for triplicates in each of three independent experiments (Student’s t -test). Significance was determined using a Student’s t -test. ( d ) Experimental scheme of RM1 Control or RM1 shCXCL16 cell implantation to CXCR6 +/+ mice for examining tumour growth and MSC cell recruitment to tumours. ( e ) The tumour growth of RM1 Control or RM1 shCXCL16 cells on CXCR6 +/+ mice was evaluated by caliper measurements over 23 days. *Significant differences between tumours grown with RM1 Control and RM1 shCXCL16 cells (mean±s.d., for n =5 animals per group, n =2 independent experiments, P <0.05; analysis of variance). ( f ) % MSCs present in RM1 Control or RM1 shCXCL16 tumours grown in CXCR6 +/+ mice (mean±s.d., for n =5 animals per group, n =2 independent experiments, Student’s t -test). Full size image Further studies examined the generation of the CAF phenotype in response to prostate cancer expressing CXCL16. In in vitro studies, MSC CXCR6+/+ cells expressed high levels of α-SMA and vimentin after treatment with conditioned media from RM1 Control cells but not after treatment with conditioned media isolated from RM1 shCXCL16 cells ( Supplementary Fig. S3a,b ). In in vivo studies, the tumours were generated from RM1 Control or RM1 shCXCL16 cells in CXCR6 +/+ mice ( Supplementary Fig. S3c ). Fewer α-SMA + and vimentin + cells were identified in tumours generated from RM1 shCXCL16 cells compared with tumours generated from RM1 Control cells ( Supplementary Fig. S3d ). Colocalization studies identified that more α-SMA + /CXCL12 + and vimentin + /CXCL12 + cells were observed in tumours from RM1 Control versus RM1 shCXCL16 cells ( Supplementary Fig. S3e,f ). CAF CXCL12 promotes prostate cancer cell EMT To explore the extent to which CXCL16 drives metastasis, we determined whether CAF-derived CXCL12 activates an EMT in prostate cancer cells ( Supplementary Fig. S4a ). Loss of cell–cell contacts and the emergence of a spindle-shaped morphology was observed following CXCL12 treatments of prostate cancer cells or when they were cocultured with MSCs CXCR6+/+ , but not when cocultured with MSC CXCR6 −/− ( Fig. 4a ). In fact, when prostate cancer cells were treated with CXCL12 or cocultured with MSCs CXCR6+/+ , but not MSCs CXCR6 −/− cells, a near complete loss of the epithelial transcriptome occurred including E-cadherin, reduced cytokeratin, enhanced expression of N-cadherin, vimentin, α-SMA, β-catenin, snail and slug were observed ( Fig. 4a–c ). When tumour microarrays were stained for E-cadherin or N-cadherin, more E-cadherin-expressing prostate cancer cells were detected in the benign prostate tissues, whereas more N-cadherin-expressing prostate cancer cells were detected in the Gleason 4+5 prostate cancers ( Fig. 4d ; Supplementary Fig. S4b ) [34] , [35] , [36] . Enhanced expression of the CXCL12 receptor CXCR4 is known to facilitate migration and metastasis in vivo [37] , [38] . We observed that CXCR4 expression by prostate cancer was enhanced following induction of an EMT phenotype in vitro and was associated with enhanced tumour growth in vivo ( Fig. 4f ). Studies with anti-CXCR4 antibody and the CXCR4 inhibitor AMD3100 showed that CXCL12 induces prostate cancer towards an EMT phenotype ( Fig. 4h ; Supplementary Fig. S4c–e ). In fact, prostate cancer cells that had undergone an EMT were significantly more responsive than their parental counterparts to CXCL12 or serum ( Fig. 5a ), such that CXCR4 blockade prevented prostate cancer migration in vitro ( Fig. 5b ). 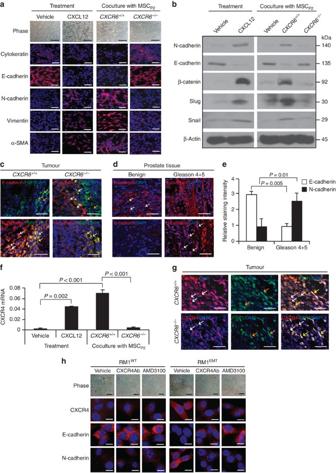Figure 4: CAF-mediated CXCL12 promotes EMT in primary tumour. (a) Vehicle-or CXCL12-treated RM1 cells, or RM1 cells cocultured with MSCs fromCXCR6+/+orCXCR6−/−mice were examined by phase contrast microscopy and immunohistochemistry (IHC) staining for cytokeratin, E-cadherin, N-cadherin, vimentin and α-SMA. Scale bars, 100 μm. Representative images from two independent studies. (b) Western blots analysis for epithelial (E-cadherin) and mesenchymal (N-cadherin, β-catenin, snail, slug) markers. Representative images from two independent studies. (c) EMT markers in the primary tumour were examined by IHC. Colocalization of E-cadherin or N-cadherin with FSP1 was observed. More E-cadherin by prostate cancer cells (red; white arrows) was detected in close proximity to FSP1-expressing MSC cells (green; orange arrows) in tumours grown inCXCR6−/−mice compared with tumours grown inCXCR6+/+mice. In contrast, more N-cadherin-expressing prostate cancer cells (red; white arrows) were detected in close proximity to N-cadherin and FSP1 co-expressing CAF cells (yellow; yellow arrows) when the tumours were grown inCXCR6+/+mice compared with tumours grown inCXCR6−/−mice. Blue, DAPI nuclear stain. Scale bars, 100 μm. Representative images derived fromn=7 mice per group. (d) IHC of E-cadherin- or N-cadherin-positive cells within benign or Gleason 4+5 prostate cancers in human prostate tissue microarrays (TMAs) (red, E-cadherin or N-cadherin, white arrows; blue, DAPI nuclear stain). Scale bars, 100 μm. (e) Quantification of paneld. Mean expression scores were multiplied by percent of positive cells in the field. Significant differences were noted between benign (n=30) or Gleason 4+5 prostate (n=6) (mean±s.d., analysis of variance). (f) CXCR4 mRNA was determined for EMT-induced RM1 cells following CXCL12 treatment or co-culture with MSCs derived fromCXCR6+/+orCXCR6−/−mice (mean±s.d.,n=3 independent experiments). (g) More CXCR4-expressing RM1 cells (red; white arrows) were detected in close proximity to CXCR4 and FSP1 (green; orange arrows) co-expressing CAF cells (yellow; yellow arrows) when the tumours were grown inCXCR6+/+mice compared with tumours grown inCXCR6−/−mice. Scale bars, 100 μm. Representative images from an experiment withn=7 animals per group. (h) AMD3100 or anti-CXCR4 antibody prevents the development of EMT by RM1 cells following CXCL12 exposure. Scale bars, 100 μm. Representative images from two independent studies. Figure 4: CAF-mediated CXCL12 promotes EMT in primary tumour. ( a ) Vehicle-or CXCL12-treated RM1 cells, or RM1 cells cocultured with MSCs from CXCR6 +/+ or CXCR6 −/− mice were examined by phase contrast microscopy and immunohistochemistry (IHC) staining for cytokeratin, E-cadherin, N-cadherin, vimentin and α-SMA. Scale bars, 100 μm. Representative images from two independent studies. ( b ) Western blots analysis for epithelial (E-cadherin) and mesenchymal (N-cadherin, β-catenin, snail, slug) markers. Representative images from two independent studies. ( c ) EMT markers in the primary tumour were examined by IHC. Colocalization of E-cadherin or N-cadherin with FSP1 was observed. More E-cadherin by prostate cancer cells (red; white arrows) was detected in close proximity to FSP1-expressing MSC cells (green; orange arrows) in tumours grown in CXCR6 −/− mice compared with tumours grown in CXCR6 +/+ mice. In contrast, more N-cadherin-expressing prostate cancer cells (red; white arrows) were detected in close proximity to N-cadherin and FSP1 co-expressing CAF cells (yellow; yellow arrows) when the tumours were grown in CXCR6 +/+ mice compared with tumours grown in CXCR6 −/− mice. Blue, DAPI nuclear stain. Scale bars, 100 μm. Representative images derived from n =7 mice per group. ( d ) IHC of E-cadherin- or N-cadherin-positive cells within benign or Gleason 4+5 prostate cancers in human prostate tissue microarrays (TMAs) (red, E-cadherin or N-cadherin, white arrows; blue, DAPI nuclear stain). Scale bars, 100 μm. ( e ) Quantification of panel d . Mean expression scores were multiplied by percent of positive cells in the field. Significant differences were noted between benign ( n =30) or Gleason 4+5 prostate ( n =6) (mean±s.d., analysis of variance). ( f ) CXCR4 mRNA was determined for EMT-induced RM1 cells following CXCL12 treatment or co-culture with MSCs derived from CXCR6 +/+ or CXCR6 −/− mice (mean±s.d., n =3 independent experiments). ( g ) More CXCR4-expressing RM1 cells (red; white arrows) were detected in close proximity to CXCR4 and FSP1 (green; orange arrows) co-expressing CAF cells (yellow; yellow arrows) when the tumours were grown in CXCR6 +/+ mice compared with tumours grown in CXCR6 −/− mice. Scale bars, 100 μm. Representative images from an experiment with n =7 animals per group. ( h ) AMD3100 or anti-CXCR4 antibody prevents the development of EMT by RM1 cells following CXCL12 exposure. Scale bars, 100 μm. Representative images from two independent studies. 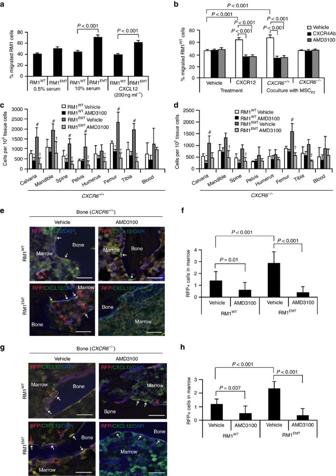Figure 5: EMT-mediated CXCR4 is highly involved in prostate cancer metastasis. (a) Migration assays were performed in Transwell plates using 10% serum or CXCL12 as chemoattractants. Migration towards 0.5% serum was used as a negative control. (b) Blockade of CXCR4 by AMD3100 or anti-CXCR4 antibody prevents prostate cancer migration towards CXCL12 or MSCs isolated fromCXCR6+/+, but notCXCR6−/−animals. Data inaandbare representative data from two independent studies (mean±s.d., analysis of variance). Significance was determined using a Student’st-test. RFP-labelled RM1WTor RM1EMTcells (Supplementary Fig. S5a) were incubated with vehicle or AMD3100in vitro, and then inoculated by intra-cardiac (i.c.) injection intoCXCR6+/+orCXCR6−/−(n=7). Metastasis was assessed by qPCR for RFP in a number of tissues. (c,d) Number of metastatic RM1 cells following i.c. injection. *Significance between RM1WTtreated with vehicle and RM1WTtreated with AMD3100 (P<0.05).#Significance between RM1WTtreated with vehicle and RM1EMTcells treated with vehicle (P<0.05).†Significance between RM1EMTtreated with vehicle and RM1EMTtreated with AMD3100 (P<0.05). Error bars represents mean±s.d.,n=2 independent experiments,P<0.05; Student’st-test. (e–h) RM1 cells expressing RFP were identified in the femur ofCXCR6+/+orCXCR6−/−mice following i.c. injection. Red arrows identify RM1 cells. White arrows identify osteoblast on the bone surface staining positive for CXCL12 expression. Scale bars, 100 μm. (f,h) Quantification of panelseandg, respectively. The numbers of RM1 cells were quantified on the endosteal region of the seven long bones. Endosteal regions were defined as 12 cell diameters from bone surfaces. (mean±s.d. (n=3), analysis of variance). Full size image Figure 5: EMT-mediated CXCR4 is highly involved in prostate cancer metastasis. ( a ) Migration assays were performed in Transwell plates using 10% serum or CXCL12 as chemoattractants. Migration towards 0.5% serum was used as a negative control. ( b ) Blockade of CXCR4 by AMD3100 or anti-CXCR4 antibody prevents prostate cancer migration towards CXCL12 or MSCs isolated from CXCR6 +/+ , but not CXCR6 −/− animals. Data in a and b are representative data from two independent studies (mean±s.d., analysis of variance). Significance was determined using a Student’s t -test. RFP-labelled RM1 WT or RM1 EMT cells ( Supplementary Fig. S5a ) were incubated with vehicle or AMD3100 in vitro , and then inoculated by intra-cardiac (i.c.) injection into CXCR6 +/+ or CXCR6 −/− ( n =7). Metastasis was assessed by qPCR for RFP in a number of tissues. ( c , d ) Number of metastatic RM1 cells following i.c. injection. *Significance between RM1 WT treated with vehicle and RM1 WT treated with AMD3100 ( P <0.05). # Significance between RM1 WT treated with vehicle and RM1 EMT cells treated with vehicle ( P <0.05). † Significance between RM1 EMT treated with vehicle and RM1 EMT treated with AMD3100 ( P <0.05). Error bars represents mean±s.d., n =2 independent experiments, P <0.05; Student’s t -test. ( e – h ) RM1 cells expressing RFP were identified in the femur of CXCR6 +/+ or CXCR6 −/− mice following i.c. injection. Red arrows identify RM1 cells. White arrows identify osteoblast on the bone surface staining positive for CXCL12 expression. Scale bars, 100 μm. ( f , h ) Quantification of panels e and g , respectively. The numbers of RM1 cells were quantified on the endosteal region of the seven long bones. Endosteal regions were defined as 12 cell diameters from bone surfaces. (mean±s.d. ( n =3), analysis of variance). Full size image EMT-induced CXCR4 expression promotes metastasis In an animal model of bone metastasis, red fluorescent protein (RFP)-expressing wild-type (RM1 WT ) or EMT-induced RM1 cells (RM1 EMT ) ( Supplementary Fig. S5a ) were incubated with AMD3100 or vehicle in vitro , and then injected by an intra-cardiac route into CXCR6 +/+ or CXCR6 −/− mice to establish prostate cancer bone metastases ( Supplementary Fig. S5b ). First, we examined CXCL12 levels in a number of osseous sites and in blood ( Supplementary Fig. S5c ). All the animals from CXCR6 +/+ or CXCR6 −/− mice had significant numbers of disseminated tumour cells (DTCs) in their bones 10 days following injection of RM1 WT or RM1 EMT cells ( Fig. 5c–h ). In contrast, RM1 WT cells pretreated with AMD3100 had a reduced number of DTCs in their calvaria, spine and femur from CXCR6 +/+ mice ( Fig. 5c ). Strikingly, animals receiving RM1 EMT cells showed a significant increase of in the total DTC load in most osseous tissues compared with animals injected with the RM1 WT cells alone. Critically, the number of DTCs were significantly reduced following CXCR4 blockade ( Fig. 5c ). However, fewer DTCs were identified in the bones of the CXCR6 −/− versus CXCR6 +/+ mice ( Fig. 5d ). Together, these data suggest that CXCL16 initiated induction of an EMT, and CXCR4 expression via MSC activation has an important and critical role in prostate cancer cell dissemination and metastasis. Tumours arise from cells that have sustained and multiple genetic mutations resulting in deregulation of normal growth-control mechanisms [39] . Recent evidence also suggests that the microenvironment itself regulates crucial neoplastic progression steps in haematological tumours [40] . Cancer cells not only interact with each other, their extracellular matrix and inflammatory cells, but also with recruited and resident cells of mesenchymal origin. The characteristic transformation of stromal cells that accompanies, or precedes the malignant conversion of epithelial cells has been linked to CAFs [41] , [42] , [43] . Several cancer types demonstrate the concept that these fibroblasts can determine the fate of the epithelial cells, promote malignant progression either through soluble factors, and cell–cell interactions and/or alterations of the extracellular matrix [43] . The complexity of these interactions has been amplified by studies showing alterations in resident cells may be drivers in cancer progression [44] . MSCs are multipotent cells that contribute to tissue homoeostasis and regeneration. Tumours recruit MSCs to facilitate tumour progression and metastasis. Here, we provide evidence that the recruitment of MSCs into prostate cancer is dependent on the expression of the CXCR6 ligand, CXCL16 by tumour cells ( Fig. 6 ). CXCR6 signalling supports the recruitment, conversion and activation of MSC into CXCL12-secreting CAFs. Moreover, enhanced CXCL12 secretion supports an EMT conversion of the prostate cancer cells and an increase in the expression of the CXCL12 receptor, CXCR4. These events result in enhanced tumour progression and ultimately extravasation and metastasis. Targeting MSCs and the CXCL16/CXCR6 axis may prevent tumour progression and metastasis of prostate cancer and provide a more effective therapeutic strategy for prostate cancer. 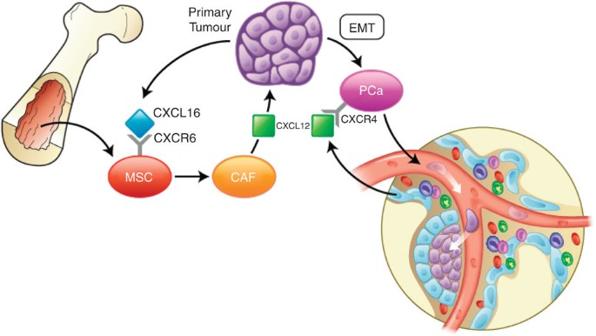Figure 6: Bone-marrow-derived MSCs promote prostate cancer growth and metastasis. Model showing potential mechanisms underlying primary prostate cancer progression by the recruitment of MSCs and bone metastasis. Secretion of CXCL16 by cancer cells recruits MSCs into tumour sites. Tumour-derived CXCL16 interacts with its receptor, CXCR6 on MSCs and activates signal transduction, leading MSCs to convert into CAFs, which secrete high levels of CXCL12. CXCL12 promotes the malignant transformation of proliferating cancer cells to an EMT. EMT enhances CXCR4 expression in prostate cancer cells. CXCR4 expression facilitates metastasis. Figure 6: Bone-marrow-derived MSCs promote prostate cancer growth and metastasis. Model showing potential mechanisms underlying primary prostate cancer progression by the recruitment of MSCs and bone metastasis. Secretion of CXCL16 by cancer cells recruits MSCs into tumour sites. Tumour-derived CXCL16 interacts with its receptor, CXCR6 on MSCs and activates signal transduction, leading MSCs to convert into CAFs, which secrete high levels of CXCL12. CXCL12 promotes the malignant transformation of proliferating cancer cells to an EMT. EMT enhances CXCR4 expression in prostate cancer cells. CXCR4 expression facilitates metastasis. Full size image Several lines of evidence demonstrate that cells with stem cell-like properties must be able to migrate into wound sites rapidly for regeneration to occur [45] , [46] , [47] , [48] . In the context of neoplasia, bone-marrow-derived MSCs have been shown to increase the metastatic potential of weakly metastatic human ovarian cancer cells, in part through the conversion to a CAF phenotype [49] . We demonstrate that primary small Lin − Sca-1 + CD45 − cells (VSEL stem cells) isolated from marrow and MSCs passaged in vitro express high mRNA levels of CXCR6 and migrate towards CXCL16. CXCL16 exists both in soluble and transmembrane forms [50] . CXCL16 is expressed on monocytes, macrophages, B cells and dendritic cells [51] , [52] , and both forms of CXCL16 are expressed by human tumour cells [15] , [16] , [22] , [53] . The precise role of soluble versus transmembrane CXCL16 in tumour progression remains unclear. Transmembrane CXCL16 may function to suppress tumour proliferation, while soluble CXCL16 induces proliferation and migration of cancer cells [19] . But which form of CXCL16 regulates prostate cancer growth within tumours is still unclear. Previous work by our group demonstrated that CXCR6 expression in tumours correlated with Gleason score. Using lentiviral vectors to overexpress CXCR6 in PC3, LNCaP C4-2B and LNCaP cells, or by reducing CXCR6 expression by siRNA, we also found that modifying CXCR6 expression altered the ability of prostate cancer cell lines to invade and grow both in vitro and in vivo [16] . In addition, CXCR6 regulates the expression of several proangiogenic factors including IL-8 and vascular endothelial growth factor, both of which are likely to participate in the regulation of tumour angiogenesis [16] . In part, binding of CXCL16 to CXCR6 induces activation of Akt, p70S6K, and eukaryotic initiation factor 4E-binding protein 1 in prostate cancer cells in addition to mammalian target of rapamycin (mTOR) pathways [16] . Moreover, rapamycin not only drastically inhibited CXCL16-induced prostate cancer cell invasion and growth but also reduced secretion of IL-8 or vascular endothelial growth factor levels and inhibited expression of other CXCR6 targets including CD44 and matrix metalloproteinase [16] . The present study further adds to the complexity of CXCL16/CXCR6 signalling and the role that paracrine/autocrine loops have in tumour progression. These findings are similar to previous observations showing that CXCL12/CXCR4 signalling [54] , [55] supports and cross-talk between CAFs and prostate cancer [33] . Our results illustrate the molecular basis for MSC recruitment into tumours and how this process leads to tumour metastasis by coupling activities of the CXCL12/CXCR4 and CXCL16/CXCR6 axes. By demonstrating that MSCs have an active role in establishing an EMT in cancer, which ultimately facilitates metastasis, MSCs are critical components of the host-response network in tumours and represent viable entities for the design of targeting therapies to prevent the establishment of distant metastasis. Animals Male CXCR6 +/+ or CXCR6 −/− mice (5–7 weeks; Jackson Laboratory, Bar Harbor, ME) and SCID mice (CB.17. SCID; Taconic, Germantown, NY) were used as transplant recipients. All animal procedures were performed in compliance with the institutional ethical requirements and approved by the University of Michigan Committee for the Use and Care of Animals (UCUCA). Cell lines The human prostate cancer cell lines PC3, LNCaP and DU145, and murine prostate cancer cell lines RM1 and Tramp were used (American Type Culture Collection, Rockville, MD). LNCaP were originally isolated from a lymph node of a patient with disseminated bony and lymph node involvement. Prostate cancer cell lines were cultured in RPMI 1640 (Invitrogen, Grand Island, NY) with 10% fetal bovine serum (FBS, Invitrogen), 1% penicillin-streptomycin (P/S, Invitrogen). The human prostate epithelial cell line RWPE-1 (ATCC) was cultured in Keratinocyte-SFM with supplements (Invitrogen). The mouse prostate epithelial cell line NMPE (CHI Scientific, Maynard, MA) was cultured in Mouse Prostate PrimaCell medium (CHI Scientific). The human breast epithelial cell line MCF-10A and breast cancer cell line MCF-7 were kindly provided by Dr Max Wicha (University of Michigan). MCF-10A cell line was cultured in DMEM/F12 with supplements (Invitrogen) and MCF-7 cell line was cultured in DMEM with supplements (Invitrogen). Conditioned media were collected and frozen after filtration through a 0.22-μm filter. For induction of EMT, RM1 cells were cultured to confluence, and serum-starved for 24 h. The cells were cultured in RPMI with 0.1% FBS supplemented with 200 ng ml −1 CXCL12 (cat. 350-NS, R&D Systems, Minneapolis, MN) for 48 h, and termed RM1 EMT versus RM1 WT . RM1 cells used in metastasis assays were labelled with RFP by lentiviral transfection ( Supplementary Fig. S5a ) and selected by FACS. MSCs Human MSCs (hMSCs, Lonza, Walkersville, MD), and freshly isolated mouse MSCs (non-passaged (P 0 )) (Lin − Sca-1 + CD45 − cells or very small embryonic-like (VSEL) stem cells) and primary bone-marrow-derived MSCs (passaged once (P 1 ) or twice (P 2 )) from CXCR6 +/+ or CXCR6 −/− mice were used for this study. The hMSCs were cultured in DMEM supplemented with 10% FBS, and 1% P/S. For mouse MSCs, after killing, marrow was flushed from femurs and tibias of both CXCR6 +/+ and CXCR6 −/− mice into α-MEM (Invitrogen) with 2% FBS to generate primary MSCs and cultured in α-MEM containing 10% FBS and 1% P/S. Once confluent, the cells were passaged 2–3 times to minimize macrophage contamination. Subsequently, repopulated bone-marrow-derived MSCs were obtained, and cells were cultured in DMEM containing 10% FBS and 1% P/S. For MSC differentiation assays, mouse primary bone-marrow-derived MSCs were cultured in adipogenic, osteogenic or chondrogenic conditions for 2 weeks, and cells were stained with Alizarin Red S, Oil Red O and Alcian Blue, respectively. Isolation of MSC P0 (VSEL) cells Small Lin − Sca-1 + CD45 − (or <8μm VSEL stem cells), referred to as MSCP 0 herein, were isolated from mononuclear bone marrow cells (1 × 10 8 cells per ml) from both CXCR6 +/+ and CXCR6 −/− mice, and resuspended in PBS containing 2% heat-inactivated FBS and 1% P/S. The cells were incubated with the following antibodies: biotin-conjugated rat anti-mouse Ly-6A/E (Sca-1) (cat. 553334, 1:50 dilution, BD Pharmingen, San Diego, CA), streptavidin-PE-Cy5 (cat. 554062, 1:50 dilution, BD Pharmingen), anti-CD45-APC (cat. 557659, 1:30 dilution, BD Pharmingen), anti-CD45R/B220-PE (cat. 553089, 1:200 dilution, BD Pharmingen), anti-Gr-1-PE (cat. 553128, 1:200 dilution, BD Pharmingen), anti-TCRαβ PE (cat. 553172, 1:200 dilution, BD Pharmingen), anti-TCRγζ PE (cat. 553178, 1:200 dilution, BD Pharmingen), anti-CD11b PE (cat. 557397, 1:200 dilution, BD Pharmingen) and anti-Ter-119 PE (cat. 553673, 1:200 dilution, BD Pharmingen). MSC P0 cells were freshly isolated by cell sorting (FACSAria II, Becton Dickinson, Mountain View, CA). Western blot analyses Cells were lysed in RIPA buffer with protease inhibitors and lysates separated on 10% SDS-polyacrylamide gel and transferred to PVDF membranes. The membranes were incubated with 5% milk for 1 h and probed overnight at 4 °C with antibodies targeting N-cadherin (cat. 610921, 1:2,500 dilution, BD Transduction laboratory, Lexington, KY), E-cadherin (cat 610181, 1:25 dilution, BD Transduction laboratory, Lexington, KY), β-catenin (cat. 9582, 1:1,000 dilution, Cell Signaling Technology, Danvers, MA), snail (cat. 3879, 1:1000 dilution, Cell Signaling), slug (cat. 9585, 1:1,000 dilution, Cell Signaling) and β-actin (cat. 4970, 1:1,000 dilution, Cell Signaling). After washing, blots were incubated with peroxidase-conjugated anti-rabbit IgG HRP secondary antibodies (cat. W401B, 1:7,500 dilution, Promega, Madison, WI) for 1 h. Protein expression was detected with SuperSignal West Pico Chemiluminescent Substrate (cat. 34080, Thermo Scientific, Rockford, IL). Immunohistochemistry Cells were fixed and tissue sections were de-waxed and re-hydrated, then blocked with Image-iT FX signal enhancer for 30 min and incubated 2 h at room temperature in dark with 10 μg ml −1 primary antibodies combined with reagents of Zenon Alexa Fluor 488 (green) or 555 (red) labelling kit. CXCR6 (cat. NLS-1102, 1:100 dilution, Novus Biologicals, Littleton, CO), fibroblast-specific protein 1 (FSP1, cat. 07-2274, 1:100 dilution, Millipore, Temecula, CA), CXCL12 (cat. ab25117, 1:100 dilution, Abcam, Cambridge, MA), cytokeratin (cat. ab9377, 1:200 dilution, Abcam), E-cadherin (cat. 610181, 1:25 dilution, BD Transduction Laboratory), N-cadherin (cat. 610921, 1:25 dilution, BD Transduction Laboratory), vimentin (cat. ab8978, 1:100 dilution, Abcam), anti-mouse α-SMA (cat. ab5694, 1:20 dilution, Abcam), CXCR4 (cat. ab2074, 1:100 dilution, Abcam) and RFP (cat. ab62341, 1:50 dilution, Abcam) antibodies were diluted in PBST (PBS plus 0.2% Triton X-100). The cells and tissue sections were post-fixed with 10% formalin for 10 min followed by processing with ProLong Gold antifade reagent with DAPI medium. Images were acquired with an Olympus FV500 confocal microscope. Human prostate tissue microarrays were purchased from US Biomax, Inc. (Rockville, MD). Anti-human CXCL16 (ab17537, 1:20 dilution, Abcam), FSP1 (cat. 07-2274, 1:100 dilution, Millipore), vimentin (cat. ab8978, 1:100 dilution, Abcam), E-cadherin (cat. 610181, 1:25 dilution, BD Transduction Laboratory) and N-cadherin (cat. 610921, 1:25 dilution, BD Transduction Laboratory) antibodies were used. Staining intensity was ranked from 1 to 4 (1, negative; 2, weak; 3, moderate; 4, strong intensity staining). Subcutaneous tumour growth Tumours were established by injecting RM1 (1 × 10 4 ) cells in growth factor-reduced Matrigel (cat. 354236, BD Bioscience, Bedford, MA) s.c. into 5- to 7-week-old male CXCR6 +/+ or CXCR6 −/− mice ( Supplementary Fig. S1h ; Supplementary Table S1 ). Tumours were also established by injecting RM1 Control or RM1 shCXCL16 (1 × 10 4 ) cells in growth factor-reduced Matrigel s.c. into 5- to 7-week-old male CXCR6 +/+ mice ( Fig. 3d ; Supplementary Table S1 ). In some cases, tumours were also established by injecting human PC3 cells (2 × 10 5 ) mixed with MSC P0 CXCR6+/+ or MSC P0 CXCR6 −/− cells (2 × 10 3 ) in growth factor-reduced Matrigel s.c. into 5- to 7-week-old male SCID mice. The animals were monitored daily and tumour volumes were evaluated every 3–7 days. Tumour volumes were calculated using the formula V= (the shortest diameter) × (the longest diameter) × height. After 23–42 days the animals were killed. The tumours were measured and prepared for Lin − Sca-1 + CD45 − cell analyses and histology. Orthotopic tumour growth After anaesthesia with 2–4% isoflurane inhalation, a low midline incision was made in the lower abdomen. The human and murine prostate cancer cells (5 × 10 4 to 5 × 10 5 ) in 20 μl of PBS were injected into the right or left dorsolateral lobe of the prostate of 5- to 7-week-old male SCID or CXCR6 +/+ mice, and the wound was closed with surgical clips. The human breast cell lines (1 × 10 6 ) in growth factor-reduced Matrigel were injected abdominal fat pad of 5–7 week-old female SCID mice ( Supplementary Fig. S1j ; Supplementary Table S1 ). In vivo metastasis assays Cells (2 × 10 5 RFP-labelled RM1 cells/mouse) were incubated with 10 μM AMD3100 (cat. A5602, Sigma) or vehicle for 30 min at 4 °C, and then introduced into 5- to 7-week-old male CXCR6 +/+ or CXCR6 −/− mice by intra-cardiac injection. qPCR and immunohistochemistry were used to identify the location of the cells. Metastasis was first assessed in osseous tissues and blood samples at day 10 by qPCR using a probe for the red fluorescent protein gene (AICSVE0-F 5′-AGAGCATCTACATGGCCAAGAAG-3′ (forward), AICSVE0-R 5′-TCGTTGTGGCTGGTGATGTC-3′ (reverse) and FAM 5′-CTTGCTGTCCACGTAGTAGT-3′ (TaqMan probe; Applied Biosystems)). The data were normalized to mouse tissue β-actin (Mm00607939_s1). Immunohistochemistry for prostate cancer cells in the marrow was also used for metastasis assays. The numbers of RM1 cells were quantified on the endosteal region of the seven long bones defined as 10 cell diameters from the bone surfaces. Statistical analyses All in vitro experiments were performed at least three times with similar results and representative assays are shown. Statistical analysis was performed by analysis of variance or Student’s t -test using GraphPad Instat (GraphPad, San Diego, CA) with significance at P <0.05. How to cite this article: Jung, Y. et al . Recruitment of mesenchymal stem cells into prostate tumours promotes metastasis. Nat. Commun. 4:1795 doi: 10.1038/ncomms2766 (2013).